Asymmetric remote C-H borylation of internal alkenes via alkene isomerization Recent years have witnessed the growing interest in the remote functionalization of alkenes for it offers a strategy to activate the challenging C–H bonds distant from the initiation point via alkene isomerization/functionalization. However, the catalytic enantioselective isomerization/functionalization with one single transition metal catalyst remains rare. Here we report a highly regio- and enantioselective cobalt-catalyzed remote C–H bond borylation of internal alkenes via sequential alkene isomerization/hydroboration. A chiral ligand featured twisted pincer, anionic, and non-rigid characters is designed and used for this transformation. This methodology, which is operationally simple using low catalyst loading without additional activator, shows excellent enantioselectivity and can be used to convert various internal alkenes with regio- and stereoisomers to valuable chiral secondary organoboronates with good functional group tolerance. Alkenes containing multiple unactivated C( sp 3 )-H bond are readily available and abundant feedstock starting materials. Catalytic asymmetric strategies based on alkenes for construction of chiral organic molecules are commonly used. Asymmetric hydrofunctionalization of unactivated alkenes via metal-hydride species has been well established for efficient construction of chiral carbon centers (Fig. 1 a) [1] , [2] , [3] . Among these transformations, alkene isomerization is considered to be a side-reaction to produce regio- and stereoisomers. However, this sequential alkene isomerization/functionalization offers an opportunity for the direct and enantioselective transformation of remote unactivated C( sp 3 )-H bonds to carbon–carbon or carbon–heteroatom bonds, which is fundamentally important and challenging for highly efficient organic synthesis (Fig. 1 b) [4] , [5] , [6] , [7] , [8] , [9] , [10] , [11] , [12] , [13] , [14] , [15] . A general pathway for the remote functionalization of alkenes via isomerization is illustrated in Fig. 1 c. Alkene 1 undergoes coordination and insertion into metal hydrogen bond to form alkyl metal species B that initiates alkene isomerization. Species B goes through β -H elimination to generate species C . After a serial of chain-walking process, a more stable alkyl metal species F , such as terminal alkyl or benzylic metal species, is formed as a terminal intermediate. Finally, species F could be trapped with a variety of reagents to afford products and regenerate catalyst, which offered a favorable thermodynamic driving force. Fig. 1 Remote functionalization of alkenes via sequential alkene isomerization/functionalization. a Asymmetric hydrofunctionalization of alkenes. b The concept of asymmetric remote functionalization of alkenes via isomerization. c A general pathway for the remote functionalization of alkenes via isomerization Full size image Recent years have witnessed the important progress in the field of catalytic alkene isomerization/functionalization with various coupling reagents [5] , [16] , such as ArX [17] , [18] , [19] , CO 2 [20] , [21] , CO/H 2 [22] , HBpin [23] , [24] , [25] , [26] , R 3 SiH [27] , [28] , [29] , and so on [11] , [30] , [31] , to afford the corresponding coupling products. Additionally, the catalytic asymmetric sequential functionalization/isomerization of alkenes terminated by oxygen-motif has been demonstrated by Sigman [32] , [33] . However, the catalytic enantioselective isomerization/functionalization with one single transition metal catalyst is restricted to only few examples [5] , [16] . Nishimura and coworkers [34] used Iridium catalyst to achieve alkene isomerization terminated by ether group and the following asymmetric hydroarylation. The development of asymmetric alkene isomerization/functionalization processes using single catalyst system is highly desirable. Chiral organoboronates are of significant utility in asymmetric synthesis for constructing a wide range of other functional groups through C-B bond transformation in a stereospecific fashion [35] , [36] . To date, several strategies [37] , such as stereospecific organoboronate homologation [38] , [39] , borylation of benzylic electrophiles [40] , [41] , asymmetric hydrogenation of alkenylboronic esters [42] , [43] , and asymmetric hydroboration of alkenes [44] , [45] , [46] , [47] , [48] , [49] , [50] , [51] , [52] , [53] , have been developed for construction of chiral secondary organoboronates. However, asymmetric hydroboration of a mixture of alkenes isomers to deliver chiral products has not been previously reported. Our group is continuously investigating asymmetric iron- or cobalt-catalyzed hydrofunctionalization of alkenes based on the ligand design [54] , [55] , [56] , [57] , [58] , [59] . Recently, we have developed a cobalt-catalyzed asymmetric sequential hydroboration/hydrogenation of internal alkynes, affording a series of chiral secondary organoboronates [56] . The control experiment demonstrated that cobalt-catalyzed asymmetric hydroboration of internal alkenes afforded secondary organoboronates with poor enantioselectivity. It would be ideal to develop a highly enantioselective cobalt-catalyzed hydroboration of internal alkenes. Here, we report a cobalt-catalyzed asymmetric remote C–H borylation of internal alkenes via isomerization/hydroboration using a imidazoline phenyl picoliamide (ImPPA) ligand with high enantioselectivity (>97% ee in most cases) (Fig. 1c ). Reaction optimization The simple internal alkene 1a was chosen as a model substrate (see Fig. 2 and Supplementary Tables 1 , 2 ). When chiral OIP ligand L1 was used [54] , the cobalt-catalyzed isomerization/hydroboration reaction of 1a with HBpin was carried out to deliver 2a in 99% yield, however, with less than 5% ee. The use of amino-derivated ligand L2 [60] or iminoaniline-derivated ligand L3 [61] led to a significant drop-off in yield, whereas the use of L2 improved the enantioselectivity to 62% ee. Using a well-defined ligand L4 [62] , the remote borylative reaction could afford 2a in 75% yield with 22% ee. Encouragingly, when ligand L5 containing a methyl group at 6-position on pyridine was used, the enantioselectivity was dramatically promoted to 88% ee. 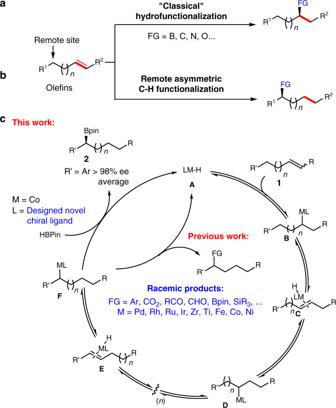Fig. 1 Remote functionalization of alkenes via sequential alkene isomerization/functionalization.aAsymmetric hydrofunctionalization of alkenes.bThe concept of asymmetric remote functionalization of alkenes via isomerization.cA general pathway for the remote functionalization of alkenes via isomerization Replacement of substituents on pyridine or oxazoline improved the enantioselectivity to 93% ee (see Supplementary Table 1 ). To our delight, the use of a more electron-rich phenyl-protected imidazoline ( L6 ) instead of oxazoline led to a significant improvement in enantioselectivity (96% ee). Assessment of various imidazolines showed that L8 with a more bulky tert -butyl group was the most effective ligand to afford 2a in 96% yield with 99% ee. Catalyst loading could be further decreased to 2.5 mol% to afford 2a in 90% yield with 98% ee. The standard conditions are identified as 1 mmol of alkene, 1.2 mmol of HBpin, 2.5 mol% of Co(OAc) 2 , 3 mol% of L8 in 1.0 mL of Et 2 O for 20 h. Fig. 2 Ligands screen for asymmetric isomerization/hydroboration. Reaction conditions: 1a (1 mmol), HBpin (1.2 mmol), Co(OAc) 2 (5.0 mol%), ligand (6.0 mol%), Et 2 O (1 M), r.t., 20 h Full size image Substrate scope With the optimized conditions in hand, we explored the scope of the olefins (Table 1 ). The cyclohexyl alkene could participate to deliver the isomerization/hydroboration product 2b in 85% yield with 96% ee. The electron-donating and electron-withdrawing groups on phenyl ring were tolerated to afford 2c – 2l in 31–84% yields with 97–>99% ee. Particularly, ortho -substituted alkene 1k could also participate in the reaction to afford 2k in 31% yield with excellent enantioselectivity (>99% ee). The alkenes containing polycyclic ring and heterocycle, such as 2-naphthyl ( 1 m ), 1-naphthyl ( 1n ), 3-pyridyl ( 1o ) and 3-benzo[ b ]thiophenyl ( 1p ), could be converted to the corresponding products 2m–2p in 64–87% yields with 97–>99% ee. Alkenes containing various functional groups, such as acetal ( 1r ), ester ( 1s ), amide ( 1t ), tertiary alcohol ( 1u ), and protected amine ( 1w ) could be tolerated to afford corresponding boronic esters in 46–71% yields with 86–99% ee. Particularly, alkene 1v with primary alcohol could also participate in the reaction and afford the product in 43% yield with 99% ee. The reaction of terminal alkene 1× with HBpin afforded a mixture of the desired product 2× with 99% ee and terminal borylated product with a b / l ratio of 1/1. The alkene with a linear undecyl group could be reacted to afford 2y in 65% yield and 98% ee with a b / l ratio of 4/1. The reactions of alkenes containing terminal tert -butyl ( 1z ) and cyclohexyl group ( 1aa ) gave the benzylic borylated products with high regio- and enantioselectivities, even walking over eight carbon–carbon bonds ( 2ab , 58% yield, 99% ee). Remarkably, the trisubstituted alkene 1ac and 1ad could also participate in the transformation to afford the corresponding products in 74% yield with 99% ee and 55% yield with >99% ee, respectively. Alkene 1ae could also be transformed to 2ae in 67% yield with 11/1 rr and 98% ee. Alkene 1af containing a disubstituted and a trisubstituted olefin has also been tested in the reaction which afforded a mixture of ( E )- 2af and ( Z )- 2af both in 94% ee. Vitamin E-derivated olefin 1ag was smoothly converted to the corresponding product 2ag in 60% yield with 98% de. Due to the unstability, some products ( 2m , 2s – 2w , 2ae–2ag ) were obtained after being directly oxidized to the corresponding alcohols. The absolute configuration was verified by comparison of the optical rotation of 2q with previously reported data and the other products were then assigned by analogy [63] . Table 1 Substrate scope of enantioselective isomerization/hydroboration of alkenes Full size table Gram-scale reaction and synthesis of bioactive molecule Notably, the preparation of 2a could be scaled up in 95% yield with 99% ee using 1 mol% of Co(OAc) 2 and 1.2 mol% of ligand (Fig. 3a ). Alkene ( 1ah ) could be transformed smoothly to afford 2ah in 80% yield with 99% ee which could easily undergo C–C bond cross-coupling in a stereospecific manner [64] to synthesize anti -breast-cancer agent 4 (Fig. 3b ). Fig. 3 Applications. a Gram-scale reaction. b Synthesis of anti -breast-cancer agent 4 Full size image Mechanistic study and other applications Cobalt-catalyzed deuterium labeling experiment was also conducted with DBpin (Fig. 4a ). Stirring a mixture of 1ai and DBpin in the presence of 5 mol% of Co(OAc) 2 and 6 mol% of L8 furnished d - 2ai with 31% d -incorporation in 2-position. Detectable amounts of deuterium were also located in the interior (3–5) positions with 69% d -incorporation in total. No deuterium was detected at benzylic positions showed that species E underwent olefin reinsertion step to prefer to form more stable benzylic cobalt species F rather than non-benzylic alkyl cobalt species. It should be note that a mixture of 1a and 1a ′ (1/1) could be transformed smoothly to a single product 2a in 95% yield with 99% ee under the standard conditions (Fig. 4b ), which demonstrated the power of this catalytic system to utilize a mixture of geometrical and positional alkene isomers. Alkenes ( E )- 1aj and ( Z )- 1aj were subjected to the reaction system and the result shows that the stereochemistry of the starting olefin has no impact on the kinetics of the reaction (see Supplementary Fig. 246 ). The reaction of product 2b under the standard conditions using ligand Ent-L7 (the enantiomer of L7 ) was conducted and no reaction occurred. The ee value of boronate 2b did not change, which indicated that the formation of the carbon boron bond was irreversible (Fig. 4c ). 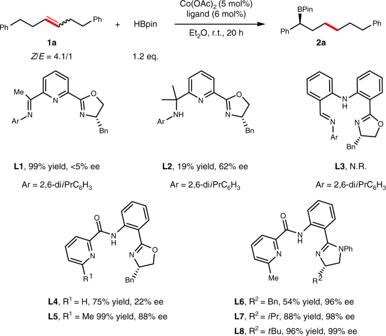Fig. 2 Ligands screen for asymmetric isomerization/hydroboration. Reaction conditions:1a(1 mmol), HBpin (1.2 mmol), Co(OAc)2(5.0 mol%), ligand (6.0 mol%), Et2O (1 M), r.t., 20 h 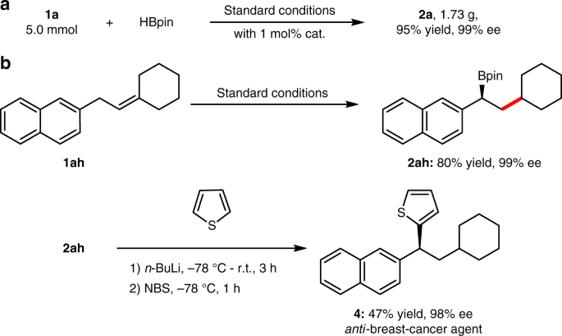Fig. 3 Applications.aGram-scale reaction.bSynthesis ofanti-breast-cancer agent4 Fig. 4 Isotope labeling and control experiments. a Deuterium labeling experiment. 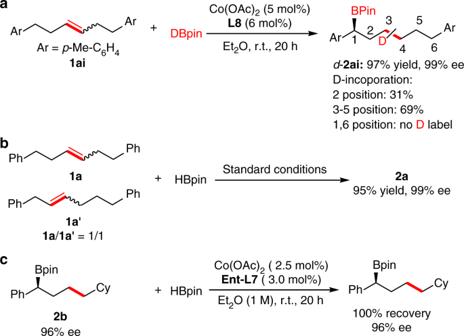Fig. 4 Isotope labeling and control experiments.aDeuterium labeling experiment.bUtilization of a mixture of geometrical and positional alkene isomers.cThe reaction of product2bwith HBpin using enantiomer ofL7 b Utilization of a mixture of geometrical and positional alkene isomers. 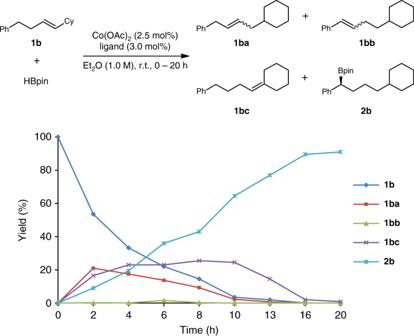Fig. 5 The time course study of1b. Reaction conditions:1b(0.5 mmol), HBpin (0.6 mmol), Co(OAc)2(2.5 mol%),L8(3.0 mol%), Et2O (1 M), r.t., 0–20 h c The reaction of product 2b with HBpin using enantiomer of L7 Full size image Time course study The time course experiment (detail see Supplementary Table 5 ) of 1b was conducted (Fig. 5 ). The observation of alkenes 1ba , 1bb , and 1bc in the process showed that the internal alkene 1b underwent a double bond walking process to both the benzylic position and cyclohexyl position. Only a small amount of the benzylic alkene 1bb (<5%) was observed during the whole process, which demonstrated that the benzylic alkyl cobalt species F might undergo a rapid σ -bond metathesis with HBpin to afford the chiral organoboronic ester 2b . Fig. 5 The time course study of 1b . Reaction conditions: 1b (0.5 mmol), HBpin (0.6 mmol), Co(OAc) 2 (2.5 mol%), L8 (3.0 mol%), Et 2 O (1 M), r.t., 0–20 h Full size image In summary, a highly regio- and enantioselective cobalt- catalyzed remote C–H bond borylation of internal alkenes via sequential alkene isomerization/hydroboration is developed. A chiral ImPPA ligand featured twisted pincer, anionic, and non-rigid characters is designed and used. This protocol is operationally simple and additional activator-free. The commonly useless mixture of internal alkenes is used for highly efficient and selective construction of valuable chiral secondary organoboronates with good functional group tolerance. The development of asymmetric transformations based on ligand design will be continuously carried out at our laboratory. Materials For NMR spectra of compounds in this manuscript, see Supplementary Figs. 1 – 204 . For HPLC spectra of compounds in this manuscript, see Supplementary Figs. 205 – 245 . For the optimization of reaction conditions and control experiments of alkene 1a , see Supplementary Tables 1 , 2 . For the experimental procedures and analytic data of compounds synthesized, see Supplementary Methods. General procedure for remote C–H borylation of internal alkenes To a 25 mL flame-dried Schlenk flask cooled under nitrogen, Co(OAc) 2 (0.025 mmol), L8 (0.03 mmol), Et 2 O (1 mL) were added. The mixture was stirred at room temperature for 5 min. Then, alkene (1.0 mmol), HBpin (180 μL, 1.2 mmol) were added in sequence and stirred at room temperature for 20 h. The resulting solution was filtered by a short pad of silica gel and washed by ether (10 mL × 2). The combined filtrate was concentrated and purified by flash column chromatography using PE/EtOAc = 20/1 as the eluent to afford the corresponding product.